Designing main-group catalysts for low-temperature methane combustion by ozone 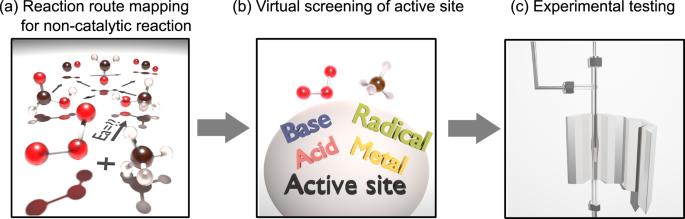Fig. 1: Rational design concept for catalytic combustion of CH4with O3. aEmploying single-component (SC)-AFIR, CH4combustion with O3was comprehensively explored to determine the key intermediates and elementary steps.bDifferent active sites were evaluated regarding the decrease inEaof the key elementary step.cHeterogeneous catalyst comprising the predicted active site was tested experimentally. The catalytic combustion of methane at a low temperature is becoming increasingly key to controlling unburned CH 4 emissions from natural gas vehicles and power plants, although the low activity of benchmark platinum-group-metal catalysts hinders its broad application. Based on automated reaction route mapping, we explore main-group elements catalysts containing Si and Al for low-temperature CH 4 combustion with ozone. Computational screening of the active site predicts that strong Brønsted acid sites are promising for methane combustion. We experimentally demonstrate that catalysts containing strong Bronsted acid sites exhibit improved CH 4 conversion at 250 °C, correlating with the theoretical predictions. The main-group catalyst (proton-type beta zeolite) delivered a reaction rate that is 442 times higher than that of a benchmark catalyst (5 wt% Pd-loaded Al 2 O 3 ) at 190 °C and exhibits higher tolerance to steam and SO 2 . Our strategy demonstrates the rational design of earth-abundant catalysts based on automated reaction route mapping. The past decades have witnessed the widespread utilization of natural gas as a clean fuel for vehicles and power plants. The catalytic combustion of methane (CH 4 ) into carbon dioxide (CO 2 ) is becoming an increasingly valuable strategy for addressing the emissions of unburned CH 4 , which exerts a greenhouse gas effect that is 22 times higher than that of CO 2 [1] , [2] , [3] . Different types of heterogeneous catalysts, such as platinum-group-metal (PGM-) [4] , [5] , [6] , [7] and metal-oxide-based catalysts [8] , [9] , [10] , have been reported. Among them, PGM-based catalysts, such as Pd- and Pt-loaded Al 2 O 3 , exhibited the highest catalytic activities [11] . However, the Pd-based catalysts suffer from high operating temperatures (>500 °C) under humidity conditions, as well as irreversible deactivation by sulfation during the co-feeding of steam and SO 2 [2] , [12] , [13] , [14] . Moreover, large amounts of PGMs (200–266 g) must be utilized to achieve the combustion of CH 4 in a natural-gas-fueled heavy-duty vehicle [15] . Additionally, the mining and purification of PGMs extensively impact the environment (the productions of 1 kg each of Pt and Pd generate 12,500 and 3880 kg of CO 2 equivalents, respectively). Conversely, the production of main-group elements generates significantly lower CO 2 equivalents (e.g., 8.2 kg of Al) [16] , [17] . Thus, it is highly desirable (economically and ecologically) to develop main-group catalysts that can function at <200 °C in the co-presence of steam and SO 2 . Conventional catalyst screening, which is based on trial-and-error experiments, may not yield discontinuous discoveries, such as the main-group-facilitated catalytic combustion of CH 4 at low temperatures. The computational reaction route mapping of the unexplored chemical reaction space can benefit the discovery of different catalytic reactions [18] , [19] , [20] , [21] , [22] , [23] . Generally, the computations of the elementary steps in combustion reactions are considered challenging because of the abundant intermediates and products that exhibit similar formation energies and activation barriers ( Ea ) [24] . To comprehensively explore the various reaction routes, density functional theory (DFT)-based automated methods for predicting reaction pathways are promising because they link the theoretical prediction to the practical designs of catalysts [25] , [26] , [27] , [28] , [29] , [30] . Maeda et al. developed an efficient automated path-searching method, namely the artificial force-induced reaction (AFIR) method, which involves pressing the atoms in given reactant molecules together by applying artificial force to form new structures (products) and assigning their transition states (TS) [30] , [31] , [32] , [33] , [34] , [35] , [36] , [37] , [38] , [39] , [40] , [41] . Via AFIR, they elucidated the entire reaction pathways of uncatalyzed reactions [32] , [37] , [39] , [40] . The automated reaction route mapping of heterogeneous catalysis systems is still formidable owing to the complexity of the surface reactions on solid materials, where the adsorption/desorption of the reactants and products, diffusion/migration of the adsorbates, and bond rearrangements proceed simultaneously [35] , [36] , [41] . Ozone (O 3 ), a strong oxidant [42] , is generated onsite by a commercial ozonizer. O 3 has been employed to enhance the catalytic performance of the gas-phase combustion of volatile organic compounds, including toluene [43] , [44] , [45] , acetone [46] , [47] , and benzene [48] , [49] . Regarding the combustion of CH 4 with O 3 [50] , [51] , [52] , zeolite-based catalysts, such as Pd [53] −, Fe [54] −, Co [55] −, and proton [56] -type zeolites, have demonstrated efficiencies at low temperatures. However, the reported studies only considered the catalytic performance; thus, the strategy for designing the catalysts based on the detailed mechanism and elementary steps must still need to be addressed. Herein, based on a computational design concept employing the AFIR method, we report a main-group catalyst for driving catalytic combustion of CH 4 with O 3 at low temperatures. First, we explored the CH 4 + O 3 reaction network toward generating CO 2 (Fig. 1a ), confirming that the formation of methanol (CH 3 OH), CH 4 + O 3 → CH 3 OH + O 2 , was the rate-determining step (RDS) of CH 4 combustion. Thereafter, we performed the virtual screening of the active sites for RDS to propose the following concept: stronger Brønsted acid sites (BASs) exhibit higher catalytic activities (Fig. 1b ). This concept was experimentally verified via CH 4 combustion tests employing O 3 at 250 °C in the presence of different BAS catalysts exhibiting different acid strengths (Fig. 1c ). Finally, we demonstrated that a proton-type beta zeolite with Si/Al = 8.5 (Hß8.5) exhibited a reaction rate that was three orders of magnitude higher than that of a PGM-based benchmark catalyst, 5 wt% Pd-loaded Al 2 O 3 (Pd5Al 2 O 3 ). The developed catalyst exhibited very high resistance to steam and SO 2 poisoning during the 170-h reaction test. Fig. 1: Rational design concept for catalytic combustion of CH 4 with O 3 . a Employing single-component (SC)-AFIR, CH 4 combustion with O 3 was comprehensively explored to determine the key intermediates and elementary steps. b Different active sites were evaluated regarding the decrease in E a of the key elementary step. c Heterogeneous catalyst comprising the predicted active site was tested experimentally. Full size image Computation of the reaction pathways toward CH 4 combustion by O 3 We explored the reaction pathway of CH 4 and O 3 (CH 4 + O 3 ) via SC-AFIR, which was an automated method for searching for reaction paths, as implemented in the GRRM program. Employing this method, the reaction routes of the non-catalytic oxidation of CH 4 into CO 2 by O 3 are automatically mapped. 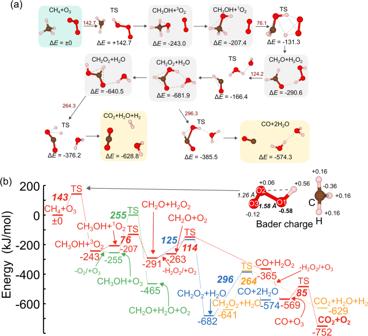Fig. 2: Result of reaction route mapping for CH4+ O3reaction without active sites. aCalculated reaction pathway of CH4+ O3, as well as the values of relative energies (ΔEs). The values written in dark red representEa.bEnergy profile of CH4combustion to yield CO2. The reaction path shown by the red lines is the most plausible for CO2formation. The result of the Bader charge analyses of the TS structures of CH4+ O3and CH3OH + O3is shown together. ΔEs are provided under each bar, and theEaare described employing the bold italic style (Unit: kJ/mol). Figure 2a shows the reaction pathways with the corresponding values of their relative energies (Δ E ) and Ea . In the first reaction, CH 4 is oxidized by O 3 to yield CH 3 OH and O 2 with strong exothermicity (243.0 kJ/mol). In the TS structure, one O atom of O 3 extracts one H atom of CH 4 to yield CH 3 and OOOH fragments, where the evaluated E a is 142.7 kJ/mol. This value is comparable to the reported experimental value for gas-phase CH 4 combustion by O 3 (148 kJ/mol) [57] . Next, the reactivity of CH 3 OH with O 3 is assessed by exploring the reaction pathway via the SC-AFIR method (see Supplementary Fig. S1 ). Although CH 3 OH is oxidized into formaldehyde (CH 2 O), H 2 O, and O 2 by O 3 , CH 3 OH + O 3 \(\to\) CH 2 O + H 2 O + O 2 , via an exothermic reaction (210.1 kJ/mol), the process requires a very high E a (255.1 kJ/mol). Alternatively, the oxidation of CH 3 OH by O 2 produces CH 2 O and H 2 O 2 , CH 3 OH + O 2 \(\to\) CH 2 O + H 2 O 2 , via a low E a of 76.1 kJ/mol (Fig. 2a ). The subsequent oxidation of CH 2 O by H 2 O 2 yields formic acid (CH 2 O 2 ) and H 2 O, CH 2 O + H 2 O 2 \(\to\) CH 2 O 2 + H 2 O, with an E a of 124.2 kJ/mol. The decomposition of the produced CH 2 O 2 yields CO 2 and H 2 , CH 2 O 2 \(\to\) CO 2 + H 2 , or CO and H 2 O molecules, CH 2 O 2 \(\to\) CO + H 2 O. However, these decomposition processes require high E a to produce CO 2 and CO (264.3 and 296.3 kJ/mol, respectively) because of the high stability of CH 2 O 2 . As an alternative reaction path, we explored the oxidation of CH 2 O by O 2 , which was abundantly present in the practical systems, via SC-AFIR (see Supplementary Fig. S2 ). Thus, the oxidation of CH 2 O by O 2 represents a facile process for producing CO and H 2 O 2 via an E a of 113.7 kJ/mol. The CO was oxidized into CO 2 + O 2 by O 3 through an E a of 84.9 kJ/mol (see Supplementary Fig. S3 ). For comparison, Nitrous oxide (N 2 O) and H 2 O 2 were assessed as alternative oxidants to oxidize CH 4 into CH 3 OH (see Supplementary Fig. S4 ). The evaluated E a of the CH 4 + N 2 O and CH 4 + H 2 O 2 reactions are 269 and 177 kJ/mol, respectively, indicating that O 3 is the most efficient oxidant for producing CH 3 OH. Fig. 2: Result of reaction route mapping for CH 4 + O 3 reaction without active sites. a Calculated reaction pathway of CH 4 + O 3 , as well as the values of relative energies (Δ E s). The values written in dark red represent E a . b Energy profile of CH 4 combustion to yield CO 2 . The reaction path shown by the red lines is the most plausible for CO 2 formation. The result of the Bader charge analyses of the TS structures of CH 4 + O 3 and CH 3 OH + O 3 is shown together. Δ E s are provided under each bar, and the E a are described employing the bold italic style (Unit: kJ/mol). Full size image Employing the explored reaction pathways (Fig. 2b ), the reaction, CH 4 + O 3 \(\to\) CH 3 OH + O 2 , was determined as the crucial process, with the highest E a in the CH 4 oxidation reaction (the RDS). To further elucidate the TS structure of this reaction, Bader charge analysis was performed to investigate the distribution of charge on each atom in the TS structure (Fig. 2b ). The total atomic charges in the CH 3 fragment are almost neutral (+0.12), indicating that it is a radical-like fragment. Regarding the OOOH fragment, the structure is divided into two parts: (I) the part comprising the H and O atoms that are closer to the CH 3 fragment (denoted as O1) and (II) that comprising the other two O atoms (denoted as O2 and O3). In the former part, the determined atomic charges of the H and O1 atoms are +0.56 and −0.58, respectively, while those of the O2 and O3 atoms in the latter part are +0.06 and −0.12, respectively. This charge distribution indicates that the OOOH fragment comprises a OH radical and O 2 molecular species. Virtual screening of catalytic sites for the reaction of CH 4 + O 3 to produce CH 3 OH + O 2 The oxidation of CH 4 by O 3 into CH 3 OH and O 2 was determined as the key reaction during CH 4 combustion (Computation of the reaction pathways toward CH4 combustion by O 3 ). To conduct the virtual screening of the catalytically active sites that effectively decrease the Ea , we carried out SC-AFIR calculations for the CH 4 + O 3 reaction on the following model active sites: (a) a Cu(0) atom as a redox site, (b) an NO molecule as a radical species, (c) pyridine (C 5 H 5 N) as a Brønsted and Lewis base site, and (d) sulfuric acid (H 2 SO 4 ) as a Brønsted acid site (Fig. 3 ). Lewis acid site is not considered here because it is known that Lewis acid sites are rapidly deactivated in the presence of H 2 O and SO 2 , which are abundantly contained in the exhaust gases and produced by the CH 4 combustion reaction. 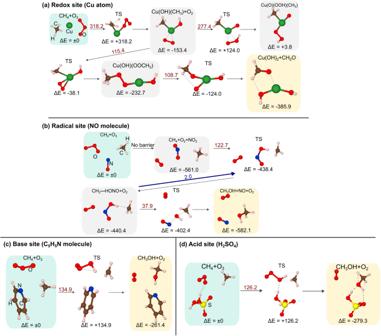Fig. 3: Result of reaction route mapping for CH4+ O3reaction on model active sites. Calculated reaction pathways of CH4+ O3onaCu(0) atom,bNO molecule,cC5H5N molecule, anddH2SO4molecule. The values of ΔEand theEa(dark red) are shown together (Unit: kJ/mol). Figure 3a shows the reaction path of CH 4 + O 3 over Cu(0). First, the C–H bond of CH 4 is cleaved by the O atom of O 3 over the Cu atom to yield OH and CH 3 groups on the Cu(II) cation (Cu(OH)(CH 3 )), as well as adsorbed O 2 molecules through a high E a (318.2 kJ/mol). Subsequently, the adsorbed O 2 molecule interacts with the neighboring CH 3 group to form CH 3 OO species on the Cu(II) cation (Cu(OH)(CH 3 OO)) via an E a of 115.4 kJ/mol, while the extraction of the H atom of the OH group (Cu(O)(OOH)(CH 3 )) is determined as an unfavorable path. Finally, the Cu(OH) 2 species and CH 2 O are produced with a moderate barrier (108.7 kJ), although the Cu(II) cation was not reduced back into the Cu(0) atom. The maximum barrier was higher than that of the uncatalyzed reaction (142.7 kJ/mol). Hence, the Cu(0) atom was not a suitable catalyst for the CH 4 + O 3 reaction. Further, the NO molecules as a representative radical site reacted with O 3 to yield O 2 and NO 2 , where the H atom of CH 4 was subsequently extracted to yield the CH 3 radical species that were bound to the nitrous acid (HONO) species (Fig. 3b ). Although the evaluated E a of this step was relatively low (122.7 kJ/mol), that of the reverse reaction (CH 3 • + HONO → CH 4 + NO 2 ) was very low (2.0 kJ/mol). Additionally, the reaction, NO 2 + CH 4 , to yield CH 3 OH + O 2 shows only a low exothermicity (−21.1 kJ/mol). These results indicate that NO is also an inefficient catalyst for the CH 4 + O 3 reaction. To compare the result above with more realistic models, the reaction route mappings on the Cu metal cluster and FeO species in ZSM-5 zeolite were carried out only for the first step of CH 4 activation (supplementally Fig. S 5 ). Note that the CH 4 activation on FeO species in ZSM-5 zeolite is known to proceed via the formation of CH 3 radical, similar to the case of the NO molecule in Fig. 3b [58] . The results indicate that, although E a for CH 4 are different, the tendency of each active site is similar (high E a of reducing back and low E a of reverse-reaction for metal and radical sites, respectively). In the case of C 5 H 5 N as a base site, O 3 slightly interacted with the basic site (the N atom) of C 5 H 5 N before reacting with CH 4 ; thus, O 3 was not decomposed by the active site (Fig. 3c ). Thereafter, CH 3 OH was produced through a similar TS structure to the gas-phase one, and the product, which was weakly bound to the base site, was slightly more stable than that in the gas phase (Δ E = − 264 kJ (on the base site) vs −243 kJ (in the gas phase)), while their E a were comparable ( E a = 134.9 vs 142.7 kJ/mol). Finally, H 2 SO 4 was assessed as an acid site. CH 3 OH was produced via an E a of 126.2 kJ/mol, which was lower than that of the gas-phase reaction (142.7 kJ/mol), with very high exothermicity (Δ E = − 279.3 kJ/mol; Fig. 3d ). As representative PGMs, Pd atom was also assessed as a potential active site for CH 4 + O 3 reaction (Supplementary Fig. S6 ). The result shows that the highest activation barrier in the reaction coordinates toward CH 2 O is 109.3 kJ/mol. Since Pd-based catalysts are known to be efficient catalysts for CH 4 combustion by O 2 , our result agrees with the previous reports [3] , [53] , [57] , [59] . Thus, the activity of Pd-based catalysts (Pd-loaded Al 2 O 3 and Pd-exchanged zeolite) for CH 4 + O 3 reaction will be experimentally tested later. Consequently, we predicted that BASs were the most effective among the virtually screened active sites for CH 4 + O 3 . In the next section, we discussed the preferable property of BAS, as well as the detailed mechanism of decreasing E a . Fig. 3: Result of reaction route mapping for CH 4 + O 3 reaction on model active sites. Calculated reaction pathways of CH 4 + O 3 on a Cu(0) atom, b NO molecule, c C 5 H 5 N molecule, and d H 2 SO 4 molecule. The values of Δ E and the E a (dark red) are shown together (Unit: kJ/mol). Full size image Promotion effect of BAS on the CH 4 + O 3 reaction We investigated the effect of the acid strength of BASs of the mineral acids on the E a of CH 4 + O 3 . H 2 SO 4 , perchloric acid (HClO 4 ), nitric acid (HNO 3 ), and phosphoric acid (H 3 PO 4 ) were evaluated as BASs exhibiting different acidities. The initial structure (IS), final structure (FS), and TS are shown in Supplementary Fig. S7 . The E a of the strong acids (128.4 and 126.2 kJ/mol for HClO 4 and H 2 SO 4 , respectively) are lower than that of the uncatalyzed reaction (142.7 kJ/mol), which is close to the value for a weak acid (142.2 and 138.8 kJ/mol for H 3 PO 4 and HNO 3 , respectively). To quantitatively evaluate the impact of the acid property, the E a of the CH 4 + O 3 reaction are plotted as a function of the stabilization energy of C 5 H 5 N on BASs ( E pyr ), as determined by DFT calculations. Notably, the adsorption of C 5 H 5 N on BAS of solid material has been widely applied to experimentally and theoretically analyze its acidity [60] , [61] , [62] . The values of E pyr for HClO 4 , H 2 SO 4 , HNO 3 , and H 3 PO 4 are −94.3, −91.1, −70.9, and −76.2 kJ/mol, respectively. This result corresponds to their experimentally obtained deprotonation enthalpies (see Supplementary Table S1 ). 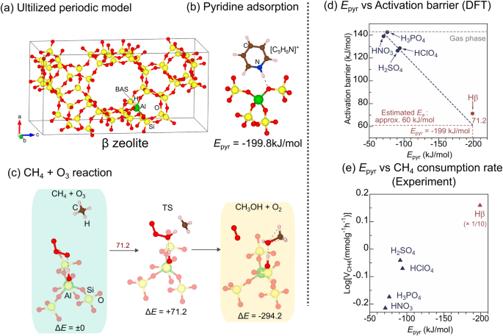Fig. 4: Theoretical and experimental evaluation for the effect of acid sites on CH4+ O3reaction. aEmployed periodic model of the ß zeolite.bStructure of the adsorption of C5H5N on BAS of ß zeolite.cTS calculations of the CH4+ O3reaction on BAS of the ß zeolite. ΔEis reported in the kJ/mol unit.Eais shown in dark red.dPlot ofEaof the CH4+ O3reaction as a function of the C5H5N-stabilization energy (Epyr) of the acids.eCH4consumption rate of the samples in 0.1% CH4+ 0.7% O3at 250 °C (He balance, total flow: 100 ml/min) as a function ofEpyr. Figure 4d shows that the E a of the CH 4 + O 3 reaction on BASs decreased with the increasing acid strengths, indicating that relatively strong BASs correspond to higher reaction rates for the CH 4 + O 3 reaction. To understand the activation mechanism within the frontier orbital theory, the projected crystal orbital Hamilton population (pCOHP) of an isolated O 3 molecule was analyzed and described in Fig. 5a . There are two anti-bonding orbitals around the Fermi level ( E F ) in the pCOHP curve of O–O bond. In the visualization of their orbitals, lower and higher energies show π* and σ* characters, respectively. Since they have anti-bonding character, it is expected that more electron charge transfer to them induces weakening of the O–O bond. 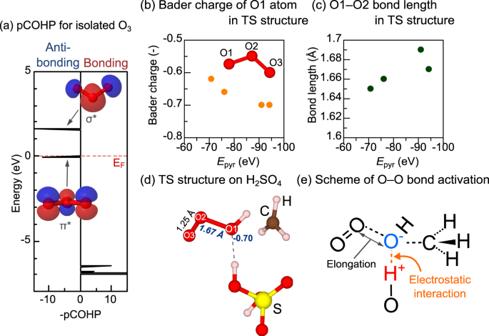Fig. 5: Theoretical interpretation of activation mechanism for CH4+ O3reaction by acid sites. aThe projected crystal orbital Hamilton population (pCOHP) curve for the O–O bond in the isolated O3molecule.bBader charge of O1 atom andcO1–O2 bond length in TS structures againstEpyr(shown in supplementary Fig.S8).dTS structure of CH4+ O3reaction over H2SO4molecule. Bader charge of O1 atom and bond lengths are shown together.eThe schematic description of O–O bond activation scheme. Figure 5b, c shows the Bader charge of O1 atom and the bond length of O1–O2 bond, respectively, against E pyr in TS structure of CH 4 + O 3 reaction (the representative TS structure is shown in Fig. 5d and others are shown in supplementary Fig. S8 ). By increasing E pyr , the charge of O1 atom increases while O1–O2 bond is elongated, indicating that the O 3 molecule was more activated on the acids with higher E pyr . A schematic description of the activation scheme is shown in Fig. 5e . By the electrostatic interaction between BAS and O1 atom, the charge transfer to O1 atom occurs, resulting in the elongation of O1–O2 bond, and thus, the BASs with high E pyr efficiently decrease the E a of CH 4 + O 3 reaction. Fig. 4: Theoretical and experimental evaluation for the effect of acid sites on CH 4 + O 3 reaction. a Employed periodic model of the ß zeolite. b Structure of the adsorption of C 5 H 5 N on BAS of ß zeolite. c TS calculations of the CH 4 + O 3 reaction on BAS of the ß zeolite. Δ E is reported in the kJ/mol unit. E a is shown in dark red. d Plot of E a of the CH 4 + O 3 reaction as a function of the C 5 H 5 N-stabilization energy ( E pyr ) of the acids. e CH 4 consumption rate of the samples in 0.1% CH 4 + 0.7% O 3 at 250 °C (He balance, total flow: 100 ml/min) as a function of E pyr . Full size image Fig. 5: Theoretical interpretation of activation mechanism for CH 4 + O 3 reaction by acid sites. a The projected crystal orbital Hamilton population (pCOHP) curve for the O–O bond in the isolated O 3 molecule. b Bader charge of O1 atom and c O1–O2 bond length in TS structures against E pyr (shown in supplementary Fig. S8 ). d TS structure of CH 4 + O 3 reaction over H 2 SO 4 molecule. Bader charge of O1 atom and bond lengths are shown together. e The schematic description of O–O bond activation scheme. Full size image Inspired by the gained insight into BASs as active sites, a proton-type zeolite (ß-type) was theoretically examined for the adsorption of C 5 H 5 N (Fig. 4a, b ). The result indicates the higher E pyr of the zeolite ( E pyr = −199.8 kJ/mol) than that of H 2 SO 4 (−91.1 kJ/mol). Note that E pyr reflects not only the strength of acidity but also the confinement effect of the zeolite cage that also probably affects the CH 4 combustion reaction [63] , [64] . The extrapolation of the linear relationship between E pyr and E a of the mineral acids indicates that the zeolite might achieve an extremely low E a (~60 kJ/mol). To verify this hypothesis, we conducted TS calculations for the CH 4 + O 3 reaction on the BAS of the zeolite. Figure 4c shows the optimized structures of IS, TS, and FS. As expected from the strong acidity of the zeolite, the computed E a (71.2 kJ/mol) is considerably lower than those for the mineral acids (126.2–142.2 kJ/mol). Next, we experimentally verified the theoretically predicted relationship between the E a and E pyr of the CH 4 + O 3 reaction. The mineral acid (3 wt% H 2 SO 4 , HClO 4 , HNO 3 , or H 3 PO 4 ) was loaded onto an SiO 2 support and tested for the reaction in a 0.1% CH 4 + 0.7% O 3 flow (total flow: 100 ml/min, He balance) at 250 °C employing a fixed-bed flow reactor (the volatility of the acid was examined by H 2 O on-off switching test; Fig. S10 ). The concentrations of CH 4 and O 3 in the outlet gas were monitored by a gas cell that was equipped with an infrared spectroscope (Supplementary Fig. S9 shows the illustration of the experimental setup). Their CH 4 conversion was maintained for 30 min. The obtained CH 4 consumption rates are plotted as a function of E pyr (Fig. 4e ). Interestingly, the observed consumption rates correlate moderately with E pyr . Next, an Hß zeolite with a relatively low Si/Al ratio (8.5) (Hß8.5) was tested via the same reaction. Therein, Hß8.5 achieves an extremely higher consumption rate than H 2 SO 4 , demonstrating the highest rate among the tested catalysts. The above results demonstrate that the high CH 4 -combustion activity of a strong BAS-based catalyst, Hß8.5, could be rationally predicted based on computational mapping of the reaction network, as well as TS calculations. In the next section (Performance of the Hß-catalyzed CH 4 combustion with O 3 ), we experimentally demonstrate the superior performance of Hß8.5 by comparing it with Pd5Al 2 O 3 as a conventional catalyst. Performance of the Hß-catalyzed CH 4 combustion with O 3 We conducted catalytic tests to experimentally demonstrate the catalytic performance of Hß8.5. 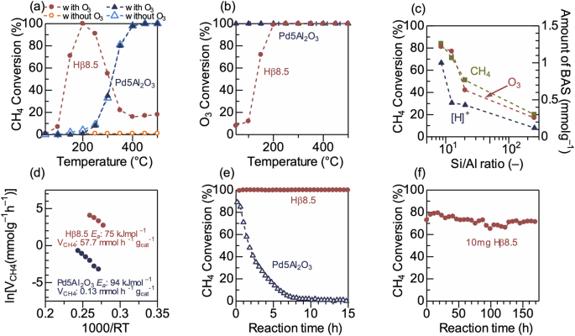Fig. 6: Catalytic test for CH4combustion reaction. aCH4andbO3conversions over 40 mg of the Hß zeolite with an Si/Al ratio of 8.5 (Hß8.5) and 40 mg of 5 wt% Pd-loaded Al2O3(Pd5Al2O3) in 0.1% CH4+ 5.95% O2+ 0.7% O3and 0.1% CH4+ 10% O2flows as functions of the reaction temperature.cConversions of CH4and O3over 40 mg of the Hß zeolite with different Si/Al ratios (8.5, 12.5, 20, and 255) in a 0.1% CH4+ 5.95% O2+ 0.7% O3flow at 150 °C, together with the amount of BAS in the ß zeolite, as evaluated via NH3-adsorption measurements.dArrhenius plots for the combustions of CH4over Hß8.5 in 0.1% CH4+ 5.95% O2+ 0.7% O3at 160–190 °C, as well as over Pd5Al2O3in 0.1% CH4+ 10% O2at 170–220 °C. The reaction rates (VCH4) at 190 °C over Hß8.5 and Pd5Al2O3are shown together (R2= 0.99 for both catalyst).eTime course of CH4conversion over 40 mg of Pd5Al2O3(at 400 °C) and Hß8.5 (at 200 °C) in 0.1% CH4+ 3% H2O + 40 ppm SO2+ 10% O2or 5.95% O2+ 0.7% O3for Pd5Al2O3and Hß8.5, respectively, with He balance (total flow: 100 ml/min).fLong-term reaction test for 10 mg of Hß8.5 in 0.1% CH4+ 5.95% O2+ 0.7% O3+ 3% H2O + 40 ppm SO2at 200 °C. Figure 6a shows the conversions of CH 4 over Hß8.5 and a benchmark catalyst (Pd5Al 2 O 3 ) in a flow of 0.1% CH 4 + 5.95% O 2 + 0.7% O 3 at different temperatures. In 0.1% CH 4 + 10% O 2 , Hß8.5 did not achieve CH 4 conversion in the entire temperature range, indicating the necessity of O 3 as the oxidant. In 0.1% CH 4 + 5.95% O 2 + 0.7% O 3 , Hß8.5 achieved the high conversion of CH 4 at 200 °C, while Pd5Al 2 O 3 required a temperature of >400 °C to achieve comparable performance. At >250 °C, the conversion of CH 4 over Hß8.5 decreased because O 3 conversion had reached 100% via self-decomposition (Fig. 5b ). To evaluate the effect of Pd loading into zeolites, Pd-exchanged ß8.5 zeolite (Pdß8.5) was prepared and then tested, resulting in low CH 4 conversion in the low-temperature region due to full decomposition of O 3 similar to the result of Pd5Al 2 O 3 (Supplementally Fig. S 11 ). The effect of BAS on the self-decomposition of O 3 into O 2 (2O 3 → 3O 2 ) was theoretically investigated because this reaction represented an obstacle to the practical application of O 3 as an oxidant. Supplementary Fig. S12 compares the optimized TS structures of the uncatalyzed and Hß-catalyzed decompositions of O 3 . The calculated E a of the uncatalyzed and Hß-catalyzed reactions are 42.3 and 69.5 kJ/mol, respectively, indicating that BAS in zeolite do not promote the self-decomposition of O 3 . This property is desirable in catalysts for CH 4 combustion by O 3 . Dissimilar to Hß8.5, Pd5Al 2 O 3 exhibited high activity toward O 3 decomposition (complete conversion even at 50 °C); hence, the addition of O 3 did not increase the CH 4 combustion activity of Pd5Al 2 O 3 . Fig. 6: Catalytic test for CH 4 combustion reaction. a CH 4 and b O 3 conversions over 40 mg of the Hß zeolite with an Si/Al ratio of 8.5 (Hß8.5) and 40 mg of 5 wt% Pd-loaded Al 2 O 3 (Pd5Al 2 O 3 ) in 0.1% CH 4 + 5.95% O 2 + 0.7% O 3 and 0.1% CH 4 + 10% O 2 flows as functions of the reaction temperature. c Conversions of CH 4 and O 3 over 40 mg of the Hß zeolite with different Si/Al ratios (8.5, 12.5, 20, and 255) in a 0.1% CH 4 + 5.95% O 2 + 0.7% O 3 flow at 150 °C, together with the amount of BAS in the ß zeolite, as evaluated via NH 3 -adsorption measurements. d Arrhenius plots for the combustions of CH 4 over Hß8.5 in 0.1% CH 4 + 5.95% O 2 + 0.7% O 3 at 160–190 °C, as well as over Pd5Al 2 O 3 in 0.1% CH 4 + 10% O 2 at 170–220 °C. The reaction rates (V CH4 ) at 190 °C over Hß8.5 and Pd5Al 2 O 3 are shown together ( R 2 = 0.99 for both catalyst). e Time course of CH 4 conversion over 40 mg of Pd5Al 2 O 3 (at 400 °C) and Hß8.5 (at 200 °C) in 0.1% CH 4 + 3% H 2 O + 40 ppm SO 2 + 10% O 2 or 5.95% O 2 + 0.7% O 3 for Pd5Al 2 O 3 and Hß8.5, respectively, with He balance (total flow: 100 ml/min). f Long-term reaction test for 10 mg of Hß8.5 in 0.1% CH 4 + 5.95% O 2 + 0.7% O 3 + 3% H 2 O + 40 ppm SO 2 at 200 °C. Full size image Figure 5c shows a plot of the conversions of CH 4 and O 3 , as well as the BAS amounts, as evaluated by NH 3 -adsorption measurement as a function of the Si/Al ratio of the utilized ß zeolites (Si/Al = 8.5, 12.5, 20, and 255). Evidently, the Al-rich ß zeolites with more BASs exhibited higher CH 4 conversions, which is consistent with the proposal from DFT calculation above. The Arrhenius plot of the Hß8.5-catalyzed CH 4 combustion with O 3 (Fig. 5d ) revealed an apparent barrier ( E a) of 75 kJ/mol, which agrees with the theoretical value of the CH 4 + O 3 reaction to yield CH 3 OH ( E a = 71.2 kJ/mol). The E a of Hß8.5 was considerably lower than that of Pd5Al 2 O 3 ( E a = 95 kJ/mol) in 0.1% CH 4 + 10% O 2 . Supplementary Fig. S13 shows the results of the kinetic analyses for estimating the reaction orders. The reaction orders of CH 4 (0.2) and O 3 (0.2) were positive. Further, the reaction rates per weight of the catalyst (for Hß8.5 and Pd5Al 2 O 3 ) for CH 4 conversion ( V CH4 ) at 190 °C were compared, and the result indicated that V CH4 of Hß8.5 (57.5 mmol h −1 g cat −1 ) was 442 times higher than that of Pd5Al 2 O 3 (0.13 mmol h −1 g cat −1 ), demonstrating that the found main-group catalyst (Hß8.5) exhibited considerably higher activity toward CH 4 combustion than the PGM-based benchmark catalyst (scientific literature on the same reaction using proton-type zeolite are limited, and thus, it is difficult to compare with the previous reports.). Further, Hß8.5 and Pd5Al 2 O 3 were tested for CH 4 combustion in the co-presence of H 2 O and SO 2 to compare their resistance to steam and SOx poisoning. Figure 5f shows the time course of CH 4 combustion over 40 mg of Hß8.5 (5.95% O 2 + 0.7% O 3 at 200 °C) and Pd5Al 2 O 3 (10% O 2 at 400 °C) in 0.1% CH 4 + 3% H 2 O + 40 ppm SO 2 . By feeding H 2 O and SO 2 , the CH 4 conversion at 400 °C over Pd5Al 2 O 3 decreased with the reaction time, reaching almost zero after 10 h. Conversely, the CH 4 conversion over Hß8.5 did not decrease at 200 °C even after 15 h, indicating that Hß8.5 was highly resistant to steam and SO 2 poisoning. Finally, 10 mg of Hß8.5 was examined for the long-term reaction test in 0.1% CH 4 + 5.95% O 2 + 0.7% O 3 + 3% H 2 O + 40 ppm SO 2 at 200 °C, and the result indicated that the catalyst did not significantly decrease the CH 4 conversion for 170 h of reaction time. To investigate the mechanism of the catalytic CH 4 combustion by O 3 in the realistic condition, ab initio molecular dynamics (AIMD) was additionally carried out for CH 4 and O 3 separately. During the simulation, the O 3 molecule frequently interacted with BASs and was present near the sites. In contrast, the CH 4 molecule diffused throughout the zeolite cage and less frequently interacted with BASs. In fact, the calculated mean diffusion coefficient of the O 3 molecule is 5.0 × 10 −4 Å 2 /fs in the simulation, while that of the CH 4 molecule is 8.4 × 10 −4 Å 2 /fs. These results indicate that, in realistic conditions, the O 3 molecule is present near BASs, and once CH 4 reaches the sites, CH 4 and O 3 react to form CH 3 OH and O 2 . In this study, we rationally designed a catalyst for low-temperature O 3 -driven catalytic combustion of CH 4 based on the elucidation of an unexplored reaction network. The CH 4 + O 3 reaction toward generating CO 2 was explored via SC-AFIR, and the formation of CH 3 OH via CH 4 + O 3 (CH 4 + O 3 → CH 3 OH + O 2 ) was determined as RDS of CH 4 combustion ( E a = 142.7 kJ/mol). To assess the various types of active sites (acid, base, redox, and radical sites), model molecules (H 2 SO 4 , C 5 H 5 N, a Cu atom, and HNO 3 ) were introduced into the system, and reaction route was calculated. Among the examined active sites, H 2 SO 4 effectively decreased the reaction ( E a = 126.2 kJ/mol); thus, different Brønsted acid catalysts with different acid strengths were examined for the TS calculation. The relationship between the acidity and calculated E a of the CH 4 + O 3 reaction (CH 3 OH formation) availed a facile catalyst design concept; the stronger the BASs afford the higher the catalytic activity. Thereafter, the theory-driven concept was experimentally verified by CH 4 combustion with O 3 at 250 °C. An Hß zeolite, which was the most effective candidate, as predicted by this concept, was experimentally tested for the CH 4 + O 3 reaction. The apparent activation energy (75 kJ/mol), which was estimated by the kinetic experiment, was consistent with the computed value (71.2 kJ/mol). Hß exhibited a very high reaction rate, which was 442 times higher than that of the benchmark catalyst, Pd5Al 2 O 3 , at 190 °C. During the catalytic tests in the presence of SO 2 and H 2 O, Hß achieved the full conversion of CH 4 at 190 °C, whereas Pd5Al 2 O 3 was completely deactivated even at a higher temperature (400 °C) owing to the poisoning of its active sites by water and SO 2 . Finally, the developed catalyst (Hß zeolite) was tested in a 170-h long-term reaction that exhibited very high resistance against water and SO 2 . In summary, O 3 , which was determined as an efficient oxidant, oxidized CH 4 into CH 3 OH as the RDS. Among the considered active sites, BAS in H 2 SO 4 molecule efficiently decreased the activation barrier of CH 3 OH formation. After stronger BASs were evaluated to be promising theoretically and experimentally, proton-type zeolite, comprising strong BASs, was experimentally tested; Hß zeolite exhibited the superior CH 4 combustion rate in the presence of O 3 . These results demonstrated that a computationally designed catalysis based on earth-abundant metal elements (Si and Al) and alternative oxidants could achieve higher activities and durabilities compared with their PGM-based ones for low-temperature CH 4 combustion. DFT calculations Spin-polarized DFT calculations were performed employing the generalized-gradient approximation of Perdew–Burke–Ernzerhof functional [65] , as implemented in the Vienna Ab Initio Simulation Package [66] , [67] (VASP), and the projected augmented waves [68] , [69] method was employed for the Kohn–Sham equations with cut-off energy of 500 eV. The Γ point was employed for the Brillouin-zone sampling [70] . DFT-D3 dispersion correction with the Becke–Johnson damping was employed for all the calculations [71] . To simulate the gas-phase reaction, calculations were conducted within a large cubic cell ( a = b = c = 15 Å). The structure of the β zeolite was obtained from the International Zeolite Association database [72] , and the lattice constants were fixed at initial values ( a = b = 12.632 Å, c = 26.186 Å, α = β = γ = 90.0°) during the calculations. The SC-AFIR method, as implemented in the GRRM17 program [38] , was applied for reaction route mapping with a model collision energy parameter of 1000 kJ/mol. Only a positive force was applied for the AFIR calculations. The H, O, and C atoms in the CH 4 and O 3 molecules were considered the targets of SC-AFIR. The locally updated plane method availed the path top points, which were subsequently optimized as TS structures and determined by the following intrinsic reaction coordinate calculation [73] . To calculate for the β zeolite, the atoms of the zeolitic framework, except for the Al atom, as well as the Si atoms adjacent to the Al and O atoms connecting to the adjacent Si, and H atoms of BAS were fixed at the crystallographic position (Fig. 4b ). The stabilization energy of C 5 H 5 N was defined, as follows: 
    E_pyr=(E_C5H5N on BAS-E_BAS-E_C5H5N)
 (1) Thus, the total energies of the models including a C 5 H 5 N molecule, acid molecules, and C 5 H 5 N interacting with the acid molecules were described as E C5H5N , E BAS , and E C5H5N on BAS , respectively. The pCOHP [74] was calculated by LOBSTER software [75] . The molecular orbitals were visualized with the VASPMO code [76] . The structures are visualized by VESTA software [77] . AIMD simulation was performed within the periodic-boundary condition as implemented in CP2K package [78] . The spin-unrestricted DFT calculation was carried out using the Perdew–Burke–Ernzerhof functional [65] within the generalized-gradient approximation. The valence electrons were described by the double-ζ valence plus polarization basis sets of the MOLOPT type [79] , and the core electrons were represented by the Goedecker–Teter–Hutter pseudopotentials [80] , [81] . The energy cutoff was set to 500 Ry. Only the Γ-point was employed for the Brillouin zone integration. The Born–Oppenheimer MD simulation was carried out with the canonical (NVT) ensemble condition using the Nóse−Hoover thermostat to control the temperature. The time step was set to 1 fs. After equilibrating for 1 ps, 50 ps of the simulation was performed for each model comprising one CH 4 or O 3 molecule, respectively. Catalysts preparations 1 g of proton-type (H) β zeolite with a Si/Al ratio of 8.5 (Hβ 8.5) was obtained via the calcination of an NH 4 + -type β zeolite that was purchased from Tosoh Co. (HSZ-920NHA) in the air at 500 °C. The 1 g of Hβ zeolites with Si/Al ratios of 20 and 255 (HSZ-940HOA and HSZ-980HOA, respectively) were supplied by Tosoh Co., and another with a Si/Al ratio of 12.5 was supplied by the Catalysis Society of Japan (JRC-Z-HΒ25). Note that the impurity of Hβ8.5 was checked by ICP measurement, and Fe, Co, Ni, Cu, and Zn were not detected (<0.01 wt%). Acid-load SiO 2 was prepared via impregnation method. 0.2 g of SiO 2 (CARiACT G–6, Fuji Silysia, S BET = ca. 500 m 2 g –1 ) was suspended in an 0.5 M aqueous solution of H 2 SO 4 , HClO 4 , H 3 PO 4 , and HNO 3 at room temperature. The water was evaporated at 50 °C from the mixture and dried in an oven at 90 °C. 1 g of Al 2 O 3 was prepared by calcining γ-AlOOH (Catapal B Alumina, Sasol) for 3 h at 900 °C. Next, 1.05 g of 5 wt% Pd-loaded Al 2 O 3 was prepared by impregnating 1 g of Al 2 O 3 with an 0.005 M aqueous HNO 3 solution Pd(NH 3 ) 2 (NO 3 ) 2 . 0.5 g of Pd-exchanged ß zeolite (Pdß8.5) was prepared by exchanging NH 4 + − ß8.5 with an 0.005 M aqueous solution of [Pd(NH 3 ) 4 ]Cl 2 at room temperature for 20 h, followed by centrifuging and washing with deionized water, drying (100 °C, 20 h), and by calcining (500 °C, 1 h, in the air). Catalytic test The catalytic test was conducted under in 0.1% CH 4 + 0.7% O 3 + 5.95% O 2 (He balance, total flow:100 ml/min) as a typical condition. 40 mg of catalyst powder was set in the fixed-bed reactor using quartz wool and the outlet was directly connected to a JASCO FT/IR-4600 spectrometer that was equipped with a triglycine sulfate (TGS) detector, in which a homemade infrared (IR) gas cell, which was equipped with KBr windows, was placed to monitor the concentrations of CH 4 and O 3 . For kinetic analysis, 5 mg of Hβ 8.5 was used to keep CH 4 conversion under 40%. The IR area of O 3 was calibrated employing an O 3 analyzer (EG-550, EcoDesign Inc.) to convert the area into concentration. To feed O 3 into the system, an O 2 flow was passed through an ozonizer (F0G-AC5G, EcoDesign Inc.) that was placed before the mainstream. The whole view of the employed setup is shown in Supplementary Fig. S9 . The NH 3 -adsorption measurement was carried out by Infrared spectroscopy (JASCO FT/IR-4200 spectrometer using a home-made in situ IR cell. The catalyst disc of the zeolite sample (40 mg,) was dehydrated under He flow at 500 °C before a background spectrum was recorded under a flow of He at 200 °C. Then, NH 3 (1%) flowed to the sample, followed by He purging before IR spectrum was taken at 200 °C. Statistics and reproducibility The experiments were not randomized.